Convergent evolution in biosynthesis of cyanogenic defence compounds in plants and insects For more than 420 million years, plants, insects and their predators have co-evolved based on a chemical arms race including deployment of refined chemical defence systems by each player. Cyanogenic glucosides are produced by numerous plants and by some specialized insects and serve an important role as defence compounds in these intimate interactions. Burnet moth larvae are able to sequester cyanogenic glucosides from their food plant as well as to carry out de novo biosynthesis. Here we show that three genes ( CYP405A2 , CYP332A3 and UGT33A1 ) encode the entire biosynthetic pathway of cyanogenic glucosides in the Burnet moth Zygaena filipendulae . In both plants and insects, convergent evolution has led to two multifunctional P450 enzymes each catalysing unusual reactions and a glucosyl-transferase acting in sequence to catalyse cyanogenic glucoside formation. Thus, plants and insects have independently found a way to package a cyanide time bomb to fend off herbivores and predators. The two cyanogenic glucosides linamarin and lotaustralin present in Zygaena species as well as in their food plant Lotus corniculatus , are derived from the amino acids valine (Val) and isoleucine (Ile), respectively. The biosynthesis of cyanogenic glucosides in plants has been elucidated and despite the numerous intermediates involved, the pathway is genetically simple in that the entire pathway is encoded by just three structural genes: two cytochromes P450 (P450) and a UDP-glycosyltransferase (UGT) [1] , [2] , [3] , [4] , [5] . Both P450s are multifunctional and catalyse unusual reactions. The first P450 catalyses two consecutive amino (N)-hydroxylations followed by a dehydration, decarboxylation and isomerization step to form a Z-oxime [6] . The second P450 catalyses dehydration and (C)-hydroxylation of the Z-oxime to produce a labile α-hydroxynitrile (cyanohydrin) [7] , which as the final step of the pathway is converted into a cyanogenic glucoside by a UGT [5] . Zygaena larvae are able to sequester linamarin and lotaustralin from their food plant L. corniculatus as well as to de novo biosynthesize the compounds depending on the level of compounds in the food plant [8] . The cyanogenic glucosides are stored in cuticular cavities in larvae [9] , and secreted on stimulation as sticky droplets to deter potential predators. Previously, the biosynthesis of linamarin and lotaustralin in Zygaena has been found to share the same intermediates as those established in plants [10] , [11] , [12] , [13] . Accordingly, the enzyme systems biosynthesizing cyanogenic glucosides in insects may have similar characteristics as those from plants [14] , but the molecular characteristics of such enzyme systems have remained unknown. To investigate whether the ability of Zygaena to de novo biosynthesize linamarin and lotaustralin represents a case of convergent or divergent evolution or is the result of horizontal gene transfer from its food plant, possible gene candidates encoding steps in the putative pathway in Zygaena have formerly been selected. Transcriptome pyrosequencing afforded ~120 P450s and 41 UGT conreads, but none of these could, from phylogenetic analyses, be assigned a function in the pathway [14] . Previous analyses of microsomes prepared from a number of different Zygaena larval tissues had shown that the ability to catalyse oxime metabolism was restricted to microsomes from the larval integument [11] . Hence, enzymes responsible for biosynthesis of linamarin and lotaustralin would be expected to be among the highly expressed proteins in integument relative to other tissues. Here we successfully expressed and characterized a number of putative candidate genes and established that three genes are necessary and sufficient to encode the enzymes catalysing the biosynthesis of linamarin and lotaustralin in Zygaena filipendulae . The genes CYP405A2 , CYP332A3 and UGT33A1 have clearly evolved convergently compared with the corresponding plant genes. Nevertheless, plants and insects have resolved the complex task of accomplishing the multistep pathway of cyanogenic glucoside synthesis in unprecedented similar ways involving the same intermediates and multifunctional P450s. Identification of candidate genes The Z. filipendulae transcriptome analysis was carried out on a larva feeding on acyanogenic food plants ( Fig. 1 ), and the larva was therefore compelled to carry out de novo biosynthesis of cyanogenic glucosides. Approximately 120 P450s and 41 UGT conreads were found in the Z. filipendulae transcriptome, and to confine the number of putative candidate genes involved in the biosynthesis of cyanogenic glucosides ( Fig. 2 ), the former pyrosequencing approach was extended with two proteomics approaches in this study. First, P450s and UGTs present in the integument microsomal fraction were identified by nano flow liquid chromatography (LC) tandem mass spectrometry (MS/MS). The LC-MS/MS data were searched against all conread sequences derived from the pyrosequencing data [14] . Among the identified proteins, 11 P450s and 5 UGTs were identified ( Supplementary Table S1 and Supplementary Data 1 and 2 ). On the basis of the overlay of proteomics and pyrosequencing data, we chose to clone ten P450s, and four UGTs. A second quantitative proteomics approach was carried out to estimate the relative abundance of the cloned P450s and UGTs in microsomal preparations from different larval tissues including haemolymph with haemocytes, gut with malphigian tubules, fatbody and integument. 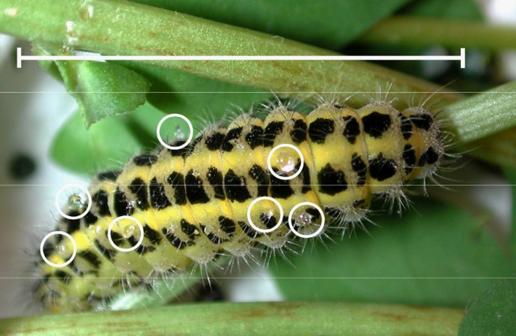Figure 1: Zygaena larva feeding on its cyanogenic host plantLotus corniculatus. The larva was stimulated to secrete defence droplets (marked by white circles) containing the two cyanogenic glucosides linamarin and lotaustralin. Scale bar, ~2 cm. The relative concentrations of the identified proteins demonstrated that the expression patterns between the individual tissues were widely different, with the integument being the tissue where most of the selected proteins were expressed highest ( Table 1 and Supplementary Data 3 ). Peaklists from the protein LC-MS/MS data used for protein identification and quantification were submitted to the PRIDE database [15] under accession codes 16842–16850. Figure 1: Zygaena larva feeding on its cyanogenic host plant Lotus corniculatus . The larva was stimulated to secrete defence droplets (marked by white circles) containing the two cyanogenic glucosides linamarin and lotaustralin. Scale bar, ~2 cm. 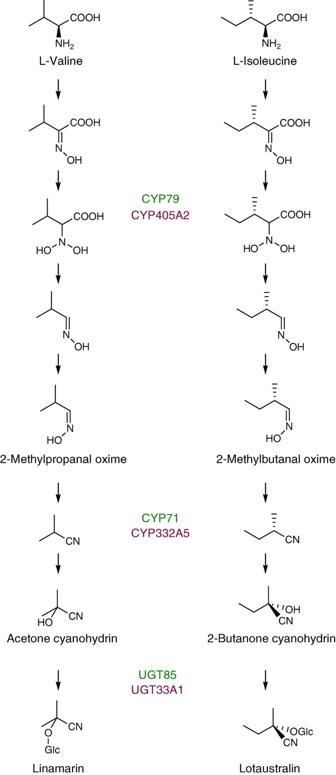Figure 2: Biosynthetic pathway of cyanogenic glucoside synthesis in plants and Zygaena. Plant (green) and Zygaena enzymes (maroon) are shown. Glc, glucose. Full size image Figure 2: Biosynthetic pathway of cyanogenic glucoside synthesis in plants and Zygaena. Plant (green) and Zygaena enzymes (maroon) are shown. Glc, glucose. Full size image Table 1 Relative concentrations of P450 and UGT proteins in different tissues of Zygaena larvae. Full size table Expression of candidate genes To identify the genes involved in the cyanogenic glucoside pathway, the selected genes were heterologously expressed in yeast. To ensure sufficient supply of reducing equivalents from nicotinamide adenine dinucleotide phosphate (NADPH) to the heterologously expressed P450s, the Z. filipendulae NADPH cytochrome P450 oxidoreductase gene ( ZfCPR ) was cloned and engineered into the genome of the expression yeast strain. All ten selected P450 s afforded the characteristic Fe 2+. CO Soret peak at 450 nm when analysed by CO-difference spectroscopy. Hence, all the selected P450s were expressed in a properly folded and active conformation ( Fig. 3a ). 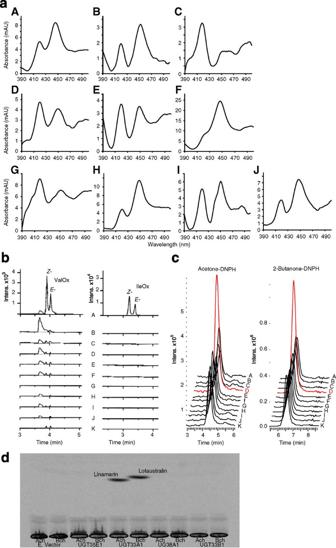Figure 3: Expression and screening results of insect cytochrome P450s and UGTs. (a) CO-difference spectra from yeast microsomes harbouring A, CYP405A2; B, CYP304F2; C, CYP405A3; D, CYP332A3; E, CYP9A36; F, CYP9A37; G, CYP6CT1; H, CYP6AE27; I, CYP4G47 and J, CYP4L17. (b) Screening of yeast microsome preparations for the ability of the P450s to convert Val/Ile into their corresponding oximes, 2-methylpropanal oxime (ValOx) and 2-methylbutanal oxime (IleOx) as monitored by SPME-GC-MS. Extracted ion chromatograms corresponding to the most abundant ion of the mass spectra for the two oximes (ValOx:m/z70; IleOx:m/z59) are shown in identical scale for all samples belonging to the respective assays. The double peaks represent the E and Z isomers of the oximes. (c) Screening of yeast microsome preparations for the ability of P450s to convert ValOx or IleOx to the corresponding cyanohydrins. Cyanohydrin formation was measured as the dissociation products acetone or 2-butanone following DNPH derivatization giving rise to acetone-DNPH and 2-butanone-DNPH monitored by LC-MS analysis. Extracted-ion chromatograms corresponding to the two adducts are shown (acetone-DNPH:m/z239; 2-butanone-DNPH:m/z253). CYP332A3 chromatograms have been highlighted in red. The background levels of acetone-DNPH and 2-butanone-DNPH originated from the omnipresence of acetone and 2-butanone in laboratory air and plastic ware. The capital letters inbandcrepresent the same P450s as inawith K being the empty vector control. (d) Screening of yeast microsomes for the ability of UGTs to convert acetone cyanohydrin (Ach) or 2-butanone cyanohydrin (Bch) into radiolabelled linamarin and lotaustralin following administration of14C-labelled UDP-glucose, and analysis of the radiolabelled products formed by thin-layer chromatography. Figure 3: Expression and screening results of insect cytochrome P450s and UGTs. ( a ) CO-difference spectra from yeast microsomes harbouring A, CYP405A2; B, CYP304F2; C, CYP405A3; D, CYP332A3; E, CYP9A36; F, CYP9A37; G, CYP6CT1; H, CYP6AE27; I, CYP4G47 and J, CYP4L17. ( b ) Screening of yeast microsome preparations for the ability of the P450s to convert Val/Ile into their corresponding oximes, 2-methylpropanal oxime (ValOx) and 2-methylbutanal oxime (IleOx) as monitored by SPME-GC-MS. Extracted ion chromatograms corresponding to the most abundant ion of the mass spectra for the two oximes (ValOx: m / z 70; IleOx: m / z 59) are shown in identical scale for all samples belonging to the respective assays. The double peaks represent the E and Z isomers of the oximes. ( c ) Screening of yeast microsome preparations for the ability of P450s to convert ValOx or IleOx to the corresponding cyanohydrins. Cyanohydrin formation was measured as the dissociation products acetone or 2-butanone following DNPH derivatization giving rise to acetone-DNPH and 2-butanone-DNPH monitored by LC-MS analysis. Extracted-ion chromatograms corresponding to the two adducts are shown (acetone-DNPH: m / z 239; 2-butanone-DNPH: m / z 253). CYP332A3 chromatograms have been highlighted in red. The background levels of acetone-DNPH and 2-butanone-DNPH originated from the omnipresence of acetone and 2-butanone in laboratory air and plastic ware. The capital letters in b and c represent the same P450s as in a with K being the empty vector control. ( d ) Screening of yeast microsomes for the ability of UGTs to convert acetone cyanohydrin (Ach) or 2-butanone cyanohydrin (Bch) into radiolabelled linamarin and lotaustralin following administration of 14 C-labelled UDP-glucose, and analysis of the radiolabelled products formed by thin-layer chromatography. Full size image Analyses of expressed proteins Microsomes prepared from yeast expressing ZfCPR and each of the ten P450s were incubated with NADPH and either Val or Ile as precursors. Of the ten P450s tested, CYP405A2 catalysed conversion of Val and Ile to their corresponding oximes, 2-methylpropanal oxime and 2-methylbutanal oxime as analysed by solid phase microextraction gas chromatography-mass spectrometry ( Fig. 3b ). Similar to cyanogenic plants, both E and Z isomer formation was observed [16] . To analyse for the conversion of oximes to cyanohydrins, the yeast microsome preparations were incubated with NADPH and 2-methylpropanal oxime or 2-methylbutanal oxime. The corresponding cyanohydrins, acetone-cyanohydrin and 2-butanone-cyanohydrin are highly labile and spontaneously decompose to cyanide and acetone or 2-butanone. To enable detection, the ketones were reacted with 2,4-dinitrophenylhydrazine (DNPH), and analysed as the corresponding hydrazones by LC-MS [17] . A background level of acetone-DNPH and 2-butanone-DNPH originating from plastic ware and the omnipresence of acetone and 2-butanone in laboratory air was detected in all samples ( Fig. 3c ). Of the ten P450 s screened, only assays with microsomes containing CYP332A3 resulted in formation of acetone-DNPH and 2-butanone-DNPH in amounts significantly above background levels. This identified CYP332A3 as the insect P450, which catalyses oxime to cyanohydrin conversion. Microsomal membrane fractions from yeast expressing the four UGTs were each incubated with 14 C-labelled UDP-glucose in combination with either acetone-cyanohydrin or 2-butanone cyanohydrin, and formation of radiolabelled products was analysed by thin-layer chromatography. Only microsomes harbouring UGT33A1 were found to catalyse glucosylation of the cyanohydrins into linamarin and lotaustralin ( Fig. 3d ). Accordingly, CYP405A2, CYP332A3 and UGT33A1 comprise the entire biosynthetic pathway of cyanogenic glucosides in Z. filipendulae ( Fig. 2 ). Phylogenetic relationships of P450s from Z. filipendulae P450s constitute one of the largest multigene families in higher eukaryotes. The genome of the reference plant Arabidopsis thaliana encodes 246, whereas 87 P450s have been identified in the silk worm ( Bombyx mori) genome. In dicotyledoneous plants similar to A. thaliana , the P450s cluster into ten monophylogetic clades designated clans. Similarly, four monophyletic clades are present in insect genomes [18] . To uncover the phylogenetic relationship of the two Zygaena P450s identified, they were included in a phylogenetic tree together with the other eight expressed Zygaena P450s and a single representative of all A. thaliana and B. mori P450 families, as well as the ten plant genes known in the cyanogenic glucoside pathway from Lotus japonicus , Sorghum bicolor , Manihot esculenta, Trifolium repens and Triglochin maritima ( Fig. 4a ). Neither CYP405 nor the CYP332 family clusters within any of the plant clans. This demonstrates that the biosynthetic pathway of cyanogenic glucosides in Zygaena has evolved by convergent evolution and not from horizontal gene transfer or divergent evolution. 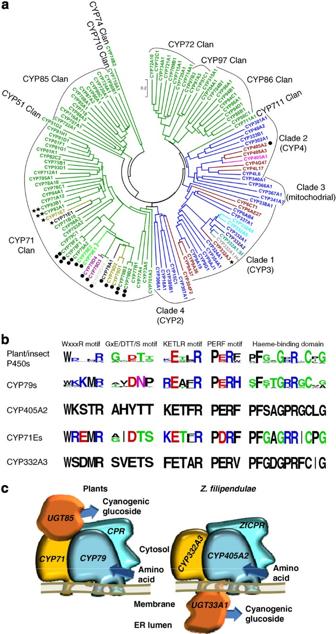Figure 4: Phylogenetic analysis of P450 genes and models of metabolon organization. (a) Neighbour joining phylogenetic tree with representatives from allA. thaliana(green) andB. mori(blue) P450 groups. Ten plant genes known from the cyanogenic glucoside pathway fromL. japonicus(purple),S. bicolor(black),M. esculenta(olive),T. repens(silver) andT. maritima(lime), as well as ten genes fromZ. filipendulae(maroon) are included. CYP405A1 fromEpiphyas postvittana(fuchsia) and CYP332s fromHelicoverpa armigera(navy),Heliothis virescens(grey),Spodoptera frugiperda(teal) andManduca sexta(aqua) are also included.•Denotes P450s known to catalyse conversion of amino acids into corresponding oximes and * denotes P450s known to catalyse metabolism of oximes.•and * represent enzymes involved in cyanogenic glucoside synthesis.••and ** represent enzymes involved in glucosinolate production. Alignment (plant–insectP450tree.mas) used for the tree can be accessed athttp://genome.ku.dk/resources/zygaena/. (b) Sequence logos of conserved regions in P450s created athttp://weblogo.berkeley.edu/logo.cgi. Plant/insect P450 sequence logos were generated from 173 insect sequences fromB. mori,Drosophila melanogaster,Anopheles gambiaeandMusca domestica, and allA. thalianasequences (excluding CYP79s). CYP79 sequence logos were generated from 12 CYP79s from plants (A. thaliana, L. japonicus, M. esculenta, S. bicolor, T. maritima) known to catalyse conversion of amino acids into corresponding oximes. CYP71E logos were generated from two CYP71Es (S. bicolor,M. esculenta) known to catalyse conversion of oximes into cyanohydrins. (c) The proposed plant metabolon, and the putative insect metabolon including the two P450s, the UGT and the CPR. In plants, the non-covalently bound UGT is thought to be anchored on the ER membrane via the P450s and with the catalytic domain facing the cytosol. In insects, the catalytic domain of the membrane bound UGT is possibly situated inside the ER lumen. If these models are correct, the cyanogenic glucoside would be liberated from the metabolon into the cytosol in plants and inside the ER lumen in insects. Figure 4: Phylogenetic analysis of P450 genes and models of metabolon organization. ( a ) Neighbour joining phylogenetic tree with representatives from all A. thaliana (green) and B. mori (blue) P450 groups. Ten plant genes known from the cyanogenic glucoside pathway from L. japonicus (purple), S. bicolor (black), M. esculenta (olive), T. repens (silver) and T. maritima (lime), as well as ten genes from Z. filipendulae (maroon) are included. CYP405A1 from Epiphyas postvittana (fuchsia) and CYP332s from Helicoverpa armigera (navy), Heliothis virescens (grey), Spodoptera frugiperda (teal) and Manduca sexta (aqua) are also included. • Denotes P450s known to catalyse conversion of amino acids into corresponding oximes and * denotes P450s known to catalyse metabolism of oximes. • and * represent enzymes involved in cyanogenic glucoside synthesis. •• and ** represent enzymes involved in glucosinolate production. Alignment (plant–insectP450tree.mas) used for the tree can be accessed at http://genome.ku.dk/resources/zygaena/ . ( b ) Sequence logos of conserved regions in P450s created at http://weblogo.berkeley.edu/logo.cgi . Plant/insect P450 sequence logos were generated from 173 insect sequences from B. mori , Drosophila melanogaster , Anopheles gambiae and Musca domestica , and all A. thaliana sequences (excluding CYP79s). CYP79 sequence logos were generated from 12 CYP79s from plants ( A. thaliana, L. japonicus, M. esculenta, S. bicolor, T. maritima ) known to catalyse conversion of amino acids into corresponding oximes. CYP71E logos were generated from two CYP71Es ( S. bicolor , M. esculenta ) known to catalyse conversion of oximes into cyanohydrins. ( c ) The proposed plant metabolon, and the putative insect metabolon including the two P450s, the UGT and the CPR. In plants, the non-covalently bound UGT is thought to be anchored on the ER membrane via the P450s and with the catalytic domain facing the cytosol. In insects, the catalytic domain of the membrane bound UGT is possibly situated inside the ER lumen. If these models are correct, the cyanogenic glucoside would be liberated from the metabolon into the cytosol in plants and inside the ER lumen in insects. Full size image We found that CYP405A2 catalysed conversion of valine and isoleucine to their corresponding oximes, and CYP332A3 catalysed oxime to cyanohydrin conversion. Furthermore, UGT33A1 catalysed glucosylation of the cyanohydrins into linamarin and lotaustralin. Consequently, CYP405A2, CYP332A3 and UGT33A1 comprise the entire biosynthetic pathway of cyanogenic glucosides in Z. filipendulae . The phylogenetic clustering of CYP405 and CYP332 families with insect P450s and not plant P450s demonstrates that the biosynthetic pathway of cyanogenic glucosides in Zygaena has evolved by convergent evolution and not from horizontal gene transfer or divergent evolution. Z. filipendulae CYP405A2 clusters within the insect CYP4 clade, which includes P450s with diverse functions ranging from xenobiotic to odorant and juvenile hormone metabolism [18] . Within the CYP4 clade, CYP405A2 clusters in a family of three CYP405A genes, two from Z. filipendulae and CYP405A1 from Epiphyas postvittana ( Fig. 4a ). The catalytic function of CYP405A1 is unknown, but most likely not identical to CYP405A2 as E. postvittana is not known to be cyanogenic [19] . Accordingly, CYP405A3 and CYP405A1 may share a yet unknown but conserved function indicating that CYP405A2 is the result of a gene duplication followed by neofunctionalization. CYP332A3 clusters in the CYP3 insect clade, which contains P450s generally involved in xenobiotic metabolism [18] . CYP332A3 clusters with six CYP332As found only in Lepidoptera species ( Fig. 4a ), and having no known function yet. CYP332A3 forms an out-group to this family, which indicates a common function of the other six CYP332As, and that CYP332A3 has been recruited from the orthologous CYP332As into the cyanogenic pathway. As the full genome of Z. filipendulae has not been sequenced, we cannot rule out that additional members of the CYP332 family are present in this species. CYP332A4 and CYP332A5 from Manduca sexta are highly expressed in the midgut [20] and a putative common function could be in detoxification of xenobiotics. Most likely, CYP332A3 has also evolved from an ancestral CYP332A involved in detoxification pathways. A parallel example in plants is the evolution of the glucosinolate synthesis pathway from the evolutionarily older cyanogenic glucoside pathway. Both pathways share the CYP79 catalysed step of amino acid to oxime conversion [21] , but in the glucosinolate pathway the subsequent steps are thought to have evolved from the general detoxification system [21] , [22] . Although the sequence identity of distantly related P450s is low, the three-dimensional structure of such P450s is quite conserved. Conserved amino acids within P450s are usually found in five motifs (WxxxR, GxE/DTT/S, KETLR, PERF and haem-binding domain) ( Fig. 4b ), in which the haem-binding domain is the most conserved [18] . The Arg in the WxxxR motif is thought to form a charge pair with the propionate group of the haem moiety. The GxE/DTT/S motif is part of the I helix, which is positioned on top of the plane of the haem. The Arg in the PERF motif forms a salt bridge with the Glu and Arg residues in the KETLR motif, and this E–R–R triad is generally thought to lock the haem pocket in the active site into the proper position and to stabilize the overall P450 core structure [23] . The haem-binding domain carries the cysteine ligand that covalently links the haem iron to the protein. In all CYP79s hitherto reported, the aromatic Phe in the PERF motif is replaced by a basic His residue ( Fig. 4b ). In addition to this unique substitution, the haem-binding domain of CYP79s is characterized by two unique Ser substitutions flanking the conserved Phe ( Fig. 4b ). In the vast majority of plant P450s, these two positions are occupied by a Phe and Gly. As the PERF and haem-binding regions are part of the active site, the polar substitutions may be related to the unusual catalytic activities of the CYP79 family catalysing N- rather than C-hydroxylations and/or to the fact that amino-acid substrates as well as several of the intermediates are hydrophilic and charged. Z. filipendulae CYP405A2 is the functional homologue to plant CYP79s, and the unique Ser substitution found in the haem motif of the plant CYP79s is also present in CYP405A2. This substantiates that a polar substitution in the haem motif is essential to enable catalysis of amino acid to oxime conversion in the biosynthesis of cyanogenic glucosides. Otherwise CYP405A2 seem to have retained many original P450 features, indicating that the evolution of plant CYP79s and CYP405A2 have followed very different paths even though they catalyse identical and complex multistep conversions. In CYP332A3, which is the functional homolog to plant CYP71Es, unique substitutions are present in the KETLR and PERF motif. In the KETLR motif, the otherwise conserved basic Arg or Lys ( Fig. 4b ) is substituted with the aromatic Phe, and in the PERF motif the conserved Phe is substituted by the much smaller Val. The latter substitution has, to our knowledge, not been observed in any other P450. Similar to CYP405A2, CYP332A3 therefore seem to have followed a different evolutionary pathway compared with plant CYP71Es. Plant and animal UGTs are phylogenetically related [24] . However, in plants the UGTs are soluble enzymes localized in the cytosol, whereas animal UGTs are generally situated in the endoplasmic reticulum (ER) membrane embedded by a C-terminal membrane anchor. The primary UGT33A1 translation product is predicted [25] , [26] to possess an N-terminal transit peptide directing the protein to the ER, in which the C-terminal membrane anchor is predicted to position the catalytic domain of the UGT33A1 in the ER lumen ( Fig. 4c ). In plants, the pathway of biosynthesis of cyanogenic glucosides is thought to be organized as a metabolon ( Fig. 4c ) to facilitate channelling of the otherwise toxic and reactive intermediates to the end product in the pathway. The metabolon is anchored within the ER membrane with the catalytic domains of the CYP79 and CYP71E facing the cytosol and the UGT non-covalently associated to the P450s [27] , [28] . Cyanogenic glucosides formed are thought to be actively transported into the vacuole by a yet unknown transporter in plants. Formation of a metabolon comprising the pathway of biosynthesis of cyanogenic glucosides in insects is to be expected from the same reasons as in plants, and several lines of evidence of specific interactions between UGTs and P450s in the mammalian detoxification system [29] , [30] support this notion. In the interaction between mammalian UGT2B7 and CYP3A4, it is not fully understood which parts of the enzymes interact, but it is speculated that the cytosolic N-terminal part of the UGT could interact with the P450. Hereby, the membrane-embedded or -associated parts of the enzymes are brought into proximity with each other in the ER membrane to facilitate channelling of the hydroxylated metabolite produced by the P450 to the UGT across the ER membrane [29] . A similar hypothetical organization of the linamarin/lotaustralin pathway in Zygaena mediated by interaction between CYP332A3 and UGT33A1 is envisioned ( Fig. 4c ). In this case, it would be the labile cyanohydrin that is channelled through the ER membrane from CYP332A3 into the immediate vicinity of the active site of UGT33A1. The orchestration of the proposed metabolon in Zygaena suggests that the formed cyanogenic glucosides are liberated inside the ER lumen ( Fig. 4c ). Thus, the transport of the cyanogenic glucoside from the integument cells into the cuticular cavities could be facilitated by exocytosis. This hypothesis is supported by the high number of Golgi complexes seen in cells adjacent to these cavities [9] . Here we report that the biosynthetic pathway of cyanogenic glucosides in Z. filipendulae is the result of convergent evolution. Only a few other pathways are known to have evolved by convergent evolution in different kingdoms. The biosynthesis of growth regulating gibberellins in higher plants and fungi [31] and syringyl lignin (S-lignin) biosynthesis in flowering plants and lycophytes [32] are examples of pathways that have evolved by convergent evolution. In gibberellin and S-lignin biosynthesis, the pathways share the same initial substrates and end products in the different organism lineages, but in each case the biosynthetic route to reach the end products differs significantly between the lineages [31] , [32] . Such differences in number of enzymes or intermediates are not observed for the cyanogenic glucoside biosynthetic pathways in insects and plants. The two pathways proceed using the same biochemical intermediates despite the significant distance between the two organisms. To our knowledge, this is the first example of biochemically identical biosynthetic pathways evolved convergently in two different kingdoms. Proteomics Zygaena larval microsomal proteins were separated by 12% SDS–polyacrylamide gel electrophoresis and stained with Coomassie blue. Two gel blocks of each lane spanning the 40–70 kDa region were excised. The gel blocks were digested with trypsin after reduction and alkylation according to ref. 33 and eluted with 0.1% trifluoroacetic acid. To identify P450s and UGTs present in the integument microsomal fraction, the peptides were analysed by reversed phase nano-high-performance liquid chromatography (HPLC), which was online hyphenated to a Q-TOF Premier (Waters) electrospray mass spectrometer. Chromatographic separation was performed by a Waters Ultimate HPLC system (Waters) fitted with a 2 cm precolumn (100 μm I.D.) and a 7 cm column of ReproSil-Pur 120 AQ-C18, 3 μm (Dr Maisch GmbH) packed in 75 μm fused silica fritted with a kasil plug and connected to a nanoelectrospray needle. The peptides were separated with a linear gradient (0–35% B in 90 min, and 35–100% B in 5 min at a flow rate of 250 nl min −1 . Solvent A was composed of 0.1% formic acid in water and solvent B was composed of 95 % acetonitrile, 0.1% formic acid and 5% water) and eluted into the electrospray ion source of the mass spectrometer operated in the positive ion V mode with data-dependent acquisition. Each MS scan was followed by four MS/MS scans of the most intense peptide ions. m / z values that had been selected for fragmentation by collision-induced dissociation were kept on an exclusion list for 60 s. MS scan times were 0.48 s, MS/MS scan times were 0.98 s and the interscan time was 0.02 s. Capillary voltage was 2 kV, cone voltage was 40 V and source temperature was 80 °C. The MS spectra were recorded from m / z 350–1500 and the MS/MS spectra from m / z 50–1500. Data of the Q-TOF Premier was processed using the MassLynxs v. 4.1 software (Waters). The resulting pkl mass lists of MS and MS/MS spectra were searched against conreads of the pyrosequencing data [14] . Both DNA sequences and translated sequences, which had been assembled and annotated to P450 protein sequences, were searched with MASCOT v. 2.2.06 hosted by an in-house server. The parameters were set as follows: specificity of trypsin: Arg and Lys, allowing two missed trypsin cleavage sites. Variable modifications: oxidation of methionine and deamidation of Asn and Gln. Fixed modification: carbamidomethyl on Cys. The peptide MS and MS/MS tolerances were set to 20 p.p.m. and 0.1 Da, respectively. To quantify the amount of selected P450s and UGTs in microsomes of the four different tissues of the larvae, peptides generated as above were undertaken phase nano-HPLC being online hyphenated to a tandem LTQ-orbitrap electrospray mass spectrometer. Chromatographic separation was performed by a Proxeon EASY-nLC system (Proxeon Biosystems) fitted with a 10 cm column of ReproSil-Pur 120 AQ-C18, 3 μm (Dr Maisch GmbH) packed in 100 μm fused silica fritted with a kasil plug and connected to a nanoelectrospray needle. The peptides were separated with a linear gradient (0–30% B in 50 min, and 30–100% B in 5 min at a flow rate of 300 nl min −1 ). Solvent A was composed of 0.1 % formic acid in water and solvent B was composed of 95% acetonitrile, 0.1% formic acid and 5% water. Mass spectra were acquired in the positive ion mode with a LTQ-Orbitrap XL (ThermoFisher) equipped with a nanoelectrospray ion source. The electrospray voltage was kept at 2.3 kV with an ion transfer temperature of 200 °C without sheath gas flow. Data-dependent acquisition was used for automated switching between MS mode in the orbitrap and MS/MS mode in the LTQ. Charges of 1,000,000 were accumulated in the LTQ before injection in the orbitrap in which a parent ion scan from m / z 300–1,800 was performed with a target peak resolution of 60,000 at m/z 400. The intensities of the MS spectra were obtained from the signal recorded during a 30 ms period in the beginning of the MS scan. The five most abundant ions with charge states above 1 and intensity above 15,000 counts were selected with an isolation width of 2.5 m / z units for MS/MS with collision-induced dissociation in the LTQ. Charges of 30,000 were accumulated, the normalized collision energy was set to 35% with activation q =0.25 and activation time 30 ms. m/z values ±10 p.p.m. of precursor ions that were selected for MS/MS were subjected to a dynamic exclusion list for 45 s. Data of the LTQ-Orbitrap were processed with MASCOT Distiller v. 2.3.2.0 software (Matrix Science) using the Orbitrap_low_res_MS2_1_opt settings as processing options. They were searched against a database of full-length protein sequences of Z. filipendulae cytochrome P450s and UGTs (CYP405A2, CYP332A3, CYP4L17, CYP9A37, CYP405A3, CYP4G47, CYP9A36, CYP6CT1, CYP304F2, CYP6AE27, UGT38A1, UGT35E1, UGT33B1, UGT33A1) using MASCOT server (version 2.2.06, Matrix Science). Search parameters were identical to the parameters stated above, except that the mass tolerance was set to 0.6 Da for MS/MS. The MASCOT Distiller quantitation package was used for quantification of proteins identified with three or more peptides. The Average protocol was used to calculate ion intensities from extracted ion chromatograms of each peptide identified with a significance threshold of P =0.05 (at least homology). Simpson's rule for numerical integration was used with survey scan as integration source. Normalization and removal of outliers were not performed. Average intensities of ion signals ascribed to the three most intense tryptic peptides for any identified protein were calculated to quantify the identified proteins as described in ref. 34 . To correct for varying amounts of proteins in the different samples, calculated protein quantities in the individual samples were normalized for the amount of protein applied to the SDS–polyacrylamide gel electrophoresis gel. Molecular biology CYP405A2 , CYP332A3 , CYP4L17 , CYP9A37 , CYP405A3 , CYP4G47 , CYP9A36 , CYP6CT1 , CYP304F2 , CYP6AE27 , UGT38A1 , UGT35E1 , UGT33B1 , UGT33A1 and ZfCPR were all amplified from Z. filipendulae cDNA using the PfuX7 polymerase [35] and subsequently cloned into the USER cassette of pYeDP60U [36] using the USER technique [37] (see Supplementary Table S2 for plasmid names and details and Supplementary Table S3 for oligonucleotides). To generate a yeast strain, which would express the ZfCPR simultaneously with the plasmid borne P450s, a ZfCPR expression cassette was integrated on the genome of the BY4741 yeast strain. The ZfCPR expression cassette from pLIFE158 was ligated into the pUC19-MGA plasmid by AvrII and FseI sites, which had been added to the ZfCPR expression cassette by PCR using oligos NB248 and NB249. Subsequently, the ZfCPR expression cassette was inserted in the yeast genome by transforming BY4741 with the 5 kbp Sbf I fragment from pLIFE0160. This linearized fragment contains the ZfCPR expression cassette and the KANMX selection gene flanked by two yeast intergenic sequences making homologous recombination possible. Positive transformants were selected for on G418 plates and correct insertion of the linearized fragment on the genome was monitored by PCR using oligonucleotides NB252, NB253, NB257, NB258 listed in Supplementary Table S3 . Biochemistry Yeast microsomal membrane fractions were prepared from 200 ml cultures grown and induced according to ref. 38 . Proper folding of the expressed P450 enzymes was monitored by CO-difference spectroscopy and functional expression of Zf CPR by cytochrome c reduction assays according to ref. 39 . All ten heterologously expressed P450 enzymes were individually tested for their ability to convert Val into 2-methylpropanal oxime and Ile into 2-methylbutanal oxime. Determination of the volatile oximes was performed by SPME GC-MS. Sampling was carried out by exposing the fibre (Supelco, 85 μm Carboxen/PDMS StableFlex, 57334-U, 'Light Blue') to the headspace from 100 μl aqueous sample solution placed at the bottom of a 1.5 ml HPLC vial. After exposure for 12 min at 80 °C with stirring, the fibre was withdrawn and fitted into the GC/MS system. This consisted of a Hewlett Packard HP5890 Series II gas chromatograph (Hewlett-Packard Company; now Agilent) hyphenated to a Jeol JMS AX505W mass spectrometer (Jeol Ltd). The capillary column was a SGE BPX (25QC2/BPX5 0.25). The head pressure was 50 kPa and the oven temperature was programmed as follows: isothermally at 50 °C for 2 min, 5 °C min −1 to 90 °C, isothermally at 90 °C for 1 min. The injector temperature was 250 °C, injection purge time 0.5 min and purge flow 15 ml helium per min. The fibre was left in the injection port during the entire GC run whereas the volatiles of the following sample were simultaneously being trapped on another fibre. Electron impact mass spectra at 70 eV were recorded in the m / z range 35–200. Presence of the two oximes was based on mass spectra comparisons with authentic standards of both oximes. All ten P450s were tested for their ability to convert oximes into their respective cyanohydrins, acetone-cyanohydrin and 2-butanone-cyanohydrin. The cyanohydrins formed are labile and dissociate into hydrogen cyanide as well as acetone or 2-butanone. The volatile ketones were trapped as 2,4-dinitrophenylhydrazones and analysed by LC-MS as described in ref. 17 . The two types of assays for P450 functionality were performed (total volume: 100 μl) using 0.2 mg microsomal protein in 20 mM Tricine pH 7.9, 1 mM NADPH, 10 mM amino acid or 0.1 mM oxime as substrate. To test the four heterologously expressed UGTs for their ability to glucosylate the cyanohydrins to produce linamarin and lotaustralin, assays were carried out using 0.2 mg microsomal protein in 20 mM Tricine pH 7.9, 10 mM aglycone and 0.02 μCi [ 14 C]-UDP-glucose. Formation of 14 C-labelled linamarin and lotaustralin was monitored by thin-layer chromatography (silica gel type 60 F 254 ) with ethyl acetate/acetone/dichlormethane/methanol/water (40:30:12:10:8) as solvent system. Phylogeny P450 sequences were aligned in MEGA4 (ref. 40 ) using CLUSTALW [41] with default settings, and refined manually. A phylogenetic Neighbor-Joining tree was generated. Accession codes: Peaklists from the protein LC-MS/MS data used for protein identification and quantification were submitted to the PRIDE database [15] under accession codes 16842, 16843, 16844, 16845, 16846, 16847, 16848, 16849 and 16850. How to cite this article: Jensen, N.B. et al . Convergent evolution in biosynthesis of cyanogenic defence compounds in plants and insects. Nat. Commun. 2:273 doi: 10.1038/ncomms1271 (2011).